Quality versus quantity of social ties in experimental cooperative networks Recent studies suggest that allowing individuals to choose their partners can help to maintain cooperation in human social networks; this behaviour can supplement behavioural reciprocity, whereby humans are influenced to cooperate by peer pressure. However, it is unknown how the rate of forming and breaking social ties affects our capacity to cooperate. Here we use a series of online experiments involving 1,529 unique participants embedded in 90 experimental networks, to show that there is a ‘Goldilocks’ effect of network dynamism on cooperation. When the rate of change in social ties is too low, subjects choose to have many ties, even if they attach to defectors. When the rate is too high, cooperators cannot detach from defectors as much as defectors re-attach and, hence, subjects resort to behavioural reciprocity and switch their behaviour to defection. Optimal levels of cooperation are achieved at intermediate levels of change in social ties. Recent theoretical attention has focused on the role that population structure might have in the emergence of cooperation [1] , [2] , [3] . This work suggests that cooperation can be maintained when individuals are situated within a social network, interacting repeatedly with their immediate neighbours. The expectation is that cooperators will form mutually reinforcing clusters, which helps them to outcompete defectors [4] , [5] , [6] . Yet, empirical work has found that static network structure has little, if any, effect on promoting cooperation [7] , [8] , [9] , [10] . In contrast, dynamic networks that allow individuals to adjust social ties are able to maintain cooperation [8] , [11] . One reason is that dynamic networks offer an additional method of responding to the past actions of others; not only can players reciprocate by strategically changing their own cooperation behaviour (thus collectively increasing or decreasing the overall levels of cooperation evinced in the group as a whole) but they can also change their network ties, engaging in ‘tie reciprocity’ [11] , [12] . Agent-based simulations show that dynamic networks favour cooperation under a wider range of assumptions about costs and benefits than static networks do [6] , [13] . As a result, there is growing interest in studying the coevolutionary dynamics of strategic behaviours and tie formation [6] , [14] , [15] , [16] , [17] . In these evolutionary models, positive feedback effects can result from preferential partner choice, where cooperative individuals keep attracting new partnerships and defecting individuals lose ties. This kind of social selection pressure can reinforce cooperation in the network, as shown by these models. However, prior theoretical work offers conflicting predictions about how cooperation will vary with the rate at which social ties may be formed or broken (the ‘rewiring rate’). Some recent theoretical (and also empirical) work shows that when individuals are allowed to rewire their networks more frequently, they are more likely to maintain cooperation [6] , [11] , [16] , [18] , suggesting that more frequent rewiring is always better. However, other work [17] suggests that too high a rewiring rate could compromise cooperation. The theorized reason is that, although very high turnover in ties helps cooperators to cut ties with defectors, it can also diminish the chance of converting such defectors into cooperators by social influence or learning [19] ; moreover, a very high turnover rate can provide relatively more opportunities for defectors to re-attach to cooperators than for cooperators to detach from defectors. Here we test these competing theoretical predictions by leveraging new tools for running economic games and conducting experiments online [20] , [21] . We find that there is a ‘Goldilocks’ effect of network dynamism on cooperation. When the rate of change in social ties is too low, subjects choose to have many ties, even if they attach to defectors; and when the rate is too high, cooperators cannot detach from defectors as much as defectors re-attach, and so subjects indeed resort to behavioural reciprocity and switch their behaviour to defection. Optimal levels of cooperation are achieved at intermediate levels of change in social ties. Structure of online experiments There is burgeoning interest in using online tools to create virtual labs to evaluate human behaviour [11] , [21] , [22] , [23] . The advantages are many, including the ability to recruit large samples quickly and the ease of conducting many replicates of experimental treatments. Using novel software and recruiting subjects from around the world to a virtual lab via the online labour market Amazon Mechanical Turk [24] , [25] , [26] , [27] , [28] , we were able to conduct a series of experiments that spanned the whole range of possible rewiring rates. We recruited 1,529 unique participants who were randomly assigned to one of nine conditions in a series of 90 realizations of our dynamic network experiments. Each participant was initially assigned a location in a random social network and then given a choice: either cooperate or defect. Participants who cooperate pay 50 units for each network neighbour and each of their neighbours receive 100 units. Participants who defect pay 0 units and their neighbours receive 0 units (each subject’s final score accumulated over all rounds was converted into dollars at an exchange rate of $1=1,000 units.) Before making each decision, participants were shown their neighbours and (after the first round) the neighbours’ previous decisions. They were only allowed to use the same strategy (cooperation or defection) simultaneously with all neighbours; this feature, of course, makes it harder to maintain cooperation because participants are more likely to use a conditional strategy and switch to defection [29] . At the end of each turn, participants were informed about the decisions of their neighbours in that round, along with their own payoff. These interactions were repeated for 15 rounds; to prevent final-round effects, we did not inform participants how many rounds would be played. Individuals were not allowed to participate in the experiment more than once (see Methods and Supplementary Fig. S1 ). Before each run of the experiment, we created a random social network with each possible connection among participants being realized with probability 0.2. Thereafter, at each round, participants chose whether or not to cooperate, and a fixed percentage of participant pairs were chosen at random in which one individual in the pair (also chosen at random) was allowed to decide whether to form a new tie if one did not exist or to cut a tie if one did exist (this percentage is the ‘rewiring rate’). In all pairs, the deciding participant was informed of the other’s choice to cooperate or defect in the preceding round. At the end of every rewiring opportunity, each participant was told the number of others who chose to break links with him or her and the number of others who formed new links with him or her. This being said, both the formation and the termination of social ties are unilateral within each round in our experiments (and different results could have been obtained if forming a new tie required mutual agreement); however, subjects can detach from newly attached alters in future rounds, when given the chance. Notably, throughout the whole experiment, our study was designed to examine how cooperation can be maintained in dynamic, evolving social networks which have roughly the same size but which were degree heterogeneous because of (preferential) partner switching. We tested nine different rewiring rates: 0, 5, 10, 30, 50, 70, 80, 90 and 100%. At higher rewiring rates, a larger fraction of the links can potentially be altered, leading to faster updating of social ties. Note that subjects were not informed of the exact rewiring rate of the sessions in which they participated. We conducted 10 experiments for each rewiring rate for a total of 90 sessions (see Methods); the average network size was 17 (s.d.=4) and there was no significant difference among rewiring rates ( P =0.35, analysis of variance). The average initial percentage of cooperative players was 65% (s.d.=11%) and there was also no significant difference among rewiring rates ( P =0.99, analysis of variance). 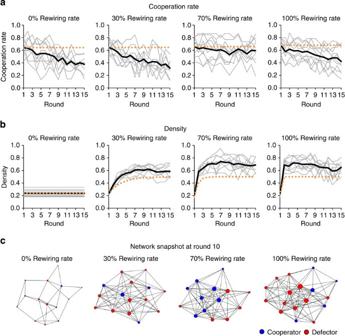Figure 1: Experimental results by rewiring rate. (a) The fraction of cooperative players by round. Light grey lines show results for each session, black lines show the average across all experimental sessions (N=10) and orange dotted lines show the initial average value. Every average line (in black) starts at a similar initial value of ~65% cooperators. Sessions with a 70% rewiring rate show the greatest maintenance of cooperation. (b) Network density (number of connections divided by maximum possible connections) by round. As a point of comparison, orange dotted lines show unbiased expectation values in networks where subjects randomly choose whether to keep or cut a tie. Densities become stable, at roughly the same level, after increasing at a speed related to the rewiring rate (larger rewiring rates are associated with more rapid convergence to a stable density). (c) Structure and strategy snapshots at round 10. Blue nodes indicate cooperators and red nodes indicate defectors. Node size is proportional to number of connections. Individual connections are shown as black lines. ‘Goldilocks’ effect of network dynamism on cooperation Figure 1a shows the cooperation rate across rounds for four of the nine rewiring rates. Whereas the slope visibly declines in the experiments with rewiring rates of 0, 30 and 100%, it remains relatively steady at the rewiring rate of 70% (see Supplementary Figs S2–S4 , and Supplementary Note 1 for the results presented in Fig. 1 ). We also examined the strategy selection data across rewiring rates using a generalized linear mixed model (GLMM) [30] with fixed effects for period and random effects for individuals. 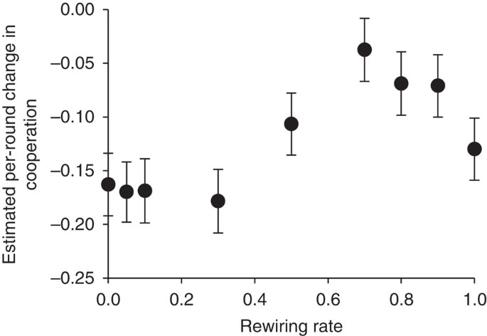Figure 2: Average change in rates of cooperation by round. Estimates based on GLMM, incorporating fixed effects for individual strategy choice and random effects for session and individual. The error bars are s.e. (N0%=161,N5%=203,N10%=165,N30%=153,N50%=184,N70%=157,N80%170,N90%=172 andN100%=179). Note that the relationship peaks at a 70% rewiring rate, suggesting that moderate rates of social change in the network (rather than low or high) are optimal for cooperation. Figure 2 shows the relationship between the network rewiring rate and cooperation. Controlling for period, there is a peak at the 70% rewiring rate ( Supplementary Table S1 ). Dynamic partner selection favours cooperation; however, at very high rewiring rates, consistent with one set of prior theoretical predictions [17] , it has an adverse effect on cooperation. Figure 1: Experimental results by rewiring rate. ( a ) The fraction of cooperative players by round. Light grey lines show results for each session, black lines show the average across all experimental sessions ( N =10) and orange dotted lines show the initial average value. Every average line (in black) starts at a similar initial value of ~65% cooperators. Sessions with a 70% rewiring rate show the greatest maintenance of cooperation. ( b ) Network density (number of connections divided by maximum possible connections) by round. As a point of comparison, orange dotted lines show unbiased expectation values in networks where subjects randomly choose whether to keep or cut a tie. Densities become stable, at roughly the same level, after increasing at a speed related to the rewiring rate (larger rewiring rates are associated with more rapid convergence to a stable density). ( c ) Structure and strategy snapshots at round 10. Blue nodes indicate cooperators and red nodes indicate defectors. Node size is proportional to number of connections. Individual connections are shown as black lines. Full size image Figure 2: Average change in rates of cooperation by round. Estimates based on GLMM, incorporating fixed effects for individual strategy choice and random effects for session and individual. The error bars are s.e. ( N 0% =161, N 5% =203, N 10% =165, N 30% =153, N 50% =184, N 70% =157, N 80% 170, N 90% =172 and N 100% =179). Note that the relationship peaks at a 70% rewiring rate, suggesting that moderate rates of social change in the network (rather than low or high) are optimal for cooperation. Full size image In these experiments, participants’ connections and strategy both change. Figure 1b shows network density, which is defined as the ratio of the number of existing connections to the number of all possible connections, for different rewiring rates. Every density (except, of course, for the 0% rewiring rate) approaches an asymptotic value between 60 and 70%, but the length of time it takes for this to happen varies by the update rate. For instance, at high rewiring rates, the density dramatically increases in the initial rounds and then stays roughly constant. We call the initial rounds the ‘pre-stable’ state and the later rounds the ‘stable’ state; we determined the number of rounds needed to transition from the pre-stable and the stable state for each rewiring rate ( Supplementary Table S2 and Supplementary Fig. S5 ). Modelling of the transition from the pre-stable to the stable state shows that sessions with a 10% rewiring rate reach a stable density at round 9, whereas sessions with 90% or 100% rewiring rates do so at the very first round ( Supplementary Fig. S4 ). Note that this transition occurs in all the rewiring rates and that this ‘stability’ is different from the rate at which ties can be rewired (which is under experimental control). Other analyses ( Supplementary Fig. S6 ) show that, by round 15, cooperators tend to have higher degree and to be more central in the network compared with defectors, across rewiring rates. Figure 1c illustrates the different appearance the networks assume, along with the greatest percentage of cooperation seen at the 70% rewiring rate. Shift from quantity to quality in partner choice The transition to the stable state appears to be related to a shift from quantity to quality in partner choice, because participants increasingly become picky about the cooperativeness of potential partners and prefer linking to cooperators rather than defectors. Note that in the various rewiring rates, the probability of choosing to connect to a defector is higher in the pre-stable state than in the stable state ( Fig. 3 ). During this initial phase in which partnerships are scarce resources, participants try to gain new connections as much as possible, whenever given the chance to do so, even agreeing to link to those who defected in the past round. However, this changes as participants acquire more ties. Participants increasingly refuse connections with defectors, and they (especially defectors) also break more existing connections with defectors. As a result, they maintain the same number of connections while attempting to increase the fraction of those connections that is with cooperators. 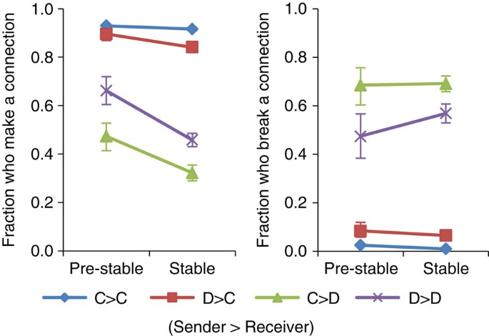Figure 3: Fraction of participants making and breaking connections. These results are grouped by behaviour: whether the ‘sender’ and ‘receiver’ of the connection cooperated or defected in the previous round. Vertical bars are s.e. (pre-stable:NmakeC>C=2,049,NmakeC>D=1,299,NmakeD>C=1,383,NmakeD>D=946,NbreakC>C=1,242,NbreakC>D=790,NbreakD>C=754 andNbreakD>D=712; stable:NmakeC>C=6,064,NmakeC>D=6,886,NmakeD>C=6,802,NmakeD>D=5,884,NbreakC>C=15,832,NbreakC>D=9,905,NbreakD>C=9,842 andNbreakD>D=10,843). Participants connect to cooperators at a constant rate, but they are less likely to make connections to defectors and more likely to break connections to defectors in the stable state, suggesting that they shift from quantity to quality over the course of the experiment. Figure 3: Fraction of participants making and breaking connections. These results are grouped by behaviour: whether the ‘sender’ and ‘receiver’ of the connection cooperated or defected in the previous round. Vertical bars are s.e. (pre-stable: N makeC>C =2,049, N makeC>D =1,299, N makeD>C =1,383, N makeD>D =946, N breakC>C =1,242, N breakC>D =790, N breakD>C =754 and N breakD>D =712; stable: N makeC>C =6,064, N makeC>D =6,886, N makeD>C =6,802, N makeD>D =5,884, N breakC>C =15,832, N breakC>D =9,905, N breakD>C =9,842 and N breakD>D =10,843). Participants connect to cooperators at a constant rate, but they are less likely to make connections to defectors and more likely to break connections to defectors in the stable state, suggesting that they shift from quantity to quality over the course of the experiment. Full size image Arms race of attachment and detachment The crucial behaviour occurs in the links between cooperators and defectors (CD links). The probability of making and breaking such links changes across rounds over the course of each session, and the relative rate of making and breaking such links varies according to the overall rewiring rate ( Fig. 4 ). At low rewiring rates, the number of newly formed CD links increases across rounds, evincing a ‘quantity-over-quality’ style of game play. As a result, cooperators increasingly become connected to defectors; this in turn increases the likelihood that a cooperator will subsequently change strategy to defection ( Fig. 5 ). At intermediate rewiring rates, the relative number of newly detached CD links rises higher than attached links across rounds, which can help cooperators to maintain their strategy and provides continuous feedback to defectors (because they are subject to detachment). However, at very high rewiring rates, cooperators who have become attached to many defectors in the initial rounds rapidly reduce their connections to defectors when given the chance to do so in later rounds. Meanwhile, defectors continue to re-attach to cooperators, which ultimately causes cooperators to switch to defection, as shown by the overall rate of cooperation declining (see Supplementary Note 2 for details). Only rewiring rates between 70% and 90% allow cooperators to keep detaching from defectors to a greater extent than the defectors can re-attach, helping to explain why cooperation is optimized in those sessions. 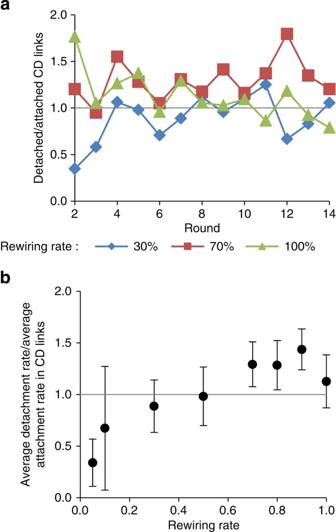Figure 4: ‘Arms race’ of making and breaking ties between cooperators and defectors. (a) Change in the ratio of detached to attached links between cooperators and defectors for low (30%), intermediate (70%), and high rewiring rates (100%). The time-averaged ratio across the full range of rewiring rates is shown inb. The error bars are s.d. (N=13). For low rewiring rates, new CD links are formed more often than existing CD links are dissolved. Cooperators become increasingly surrounded by defectors as a result, and cooperation in the group declines. At intermediate rewiring rates (for example, 70%), cooperators can more effectively shun defectors and, thus, cooperation is maintained in the group. At a 100% rewiring rate, however, the detachment rate drops compared with the attachment rate, which explains why cooperation is optimized in those sessions. Figure 4: ‘Arms race’ of making and breaking ties between cooperators and defectors. ( a ) Change in the ratio of detached to attached links between cooperators and defectors for low (30%), intermediate (70%), and high rewiring rates (100%). The time-averaged ratio across the full range of rewiring rates is shown in b . The error bars are s.d. ( N =13). For low rewiring rates, new CD links are formed more often than existing CD links are dissolved. Cooperators become increasingly surrounded by defectors as a result, and cooperation in the group declines. At intermediate rewiring rates (for example, 70%), cooperators can more effectively shun defectors and, thus, cooperation is maintained in the group. At a 100% rewiring rate, however, the detachment rate drops compared with the attachment rate, which explains why cooperation is optimized in those sessions. 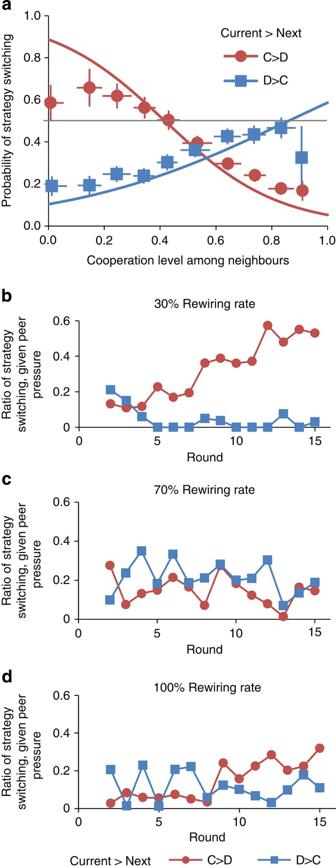Figure 5: Intermediate network rewiring rates promote reciprocal cooperation. (a) The probability of subjects switching their current strategy depends on cooperation levels among their neighbours. The dots are expectation values, the error bars represent 95% confidence intervals, and the solid lines are the estimated probability functions by GLMM incorporating random effects for sessions and individuals (red line:N=10,866,P<0.01; blue line:N=9,341,P<0.01). The intersections between the horizontal line and the estimated probability lines mark the threshold level of cooperation among neighbours at which individuals switch their current strategies with 50% chance. Cooperators are more likely to change to defection when the cooperation ratio among neighbours is >41.7%, whereas defectors are more likely to change to cooperating when the cooperation ratio among neighbours exceeds 86.0%. Panelsb–dshow how the fractions of subjects who are more likely to switch to the opposite strategies change with respect to game rounds for different rewiring rates of 30%, 70%, and 100%, respectively. The arms race of attachment and detachment, as shown inFig. 4, has an impact on strategy updates of subjects; only at intermediate rewiring rates does the proportion of defectors who are more likely to switch to cooperation exceed that of cooperators more likely to switch to defection. Full size image Figure 5: Intermediate network rewiring rates promote reciprocal cooperation. ( a ) The probability of subjects switching their current strategy depends on cooperation levels among their neighbours. The dots are expectation values, the error bars represent 95% confidence intervals, and the solid lines are the estimated probability functions by GLMM incorporating random effects for sessions and individuals (red line: N =10,866, P <0.01; blue line: N =9,341, P <0.01). The intersections between the horizontal line and the estimated probability lines mark the threshold level of cooperation among neighbours at which individuals switch their current strategies with 50% chance. Cooperators are more likely to change to defection when the cooperation ratio among neighbours is >41.7%, whereas defectors are more likely to change to cooperating when the cooperation ratio among neighbours exceeds 86.0%. Panels b – d show how the fractions of subjects who are more likely to switch to the opposite strategies change with respect to game rounds for different rewiring rates of 30%, 70%, and 100%, respectively. The arms race of attachment and detachment, as shown in Fig. 4 , has an impact on strategy updates of subjects; only at intermediate rewiring rates does the proportion of defectors who are more likely to switch to cooperation exceed that of cooperators more likely to switch to defection. Full size image Our findings comport with one set of theoretical results that counterintuitively predict that cooperation will not rise monotonically with dynamism in the network [17] . It is not where the actual peak occurs (at 70% in the present study) that is important here, but rather the fact that the overall curve has a parabolic shape. There is a kind of arms race of attaching and detaching between cooperators and defectors that affects actors’ cooperative behaviour. The achievement of a maximum level of cooperation in the group at an intermediate rewiring rate can be understood as follows. Under low rewiring rates, cooperators at times unselectively attach to and/or fail to detach from defectors, presumably in the hope that these defectors would, via behavioural reciprocity, be converted into cooperators and reciprocate in later rounds. Defectors, on the other hand, almost always capitalize on rewiring opportunities exclusively to attach to cooperators ( Fig. 3 ). Still, defectors are unavoidably faced with the threat of losing existing ties, whereas some cooperators keep gaining new ties. This feedback helps to maintain cooperation in dynamic social networks. As the rewiring rate rises above a threshold (~70% in the present study), however, cooperators are increasingly overwhelmed by defectors who persistently chase after them. Thus, at very high rewiring rates (for instance, at a 100% rewiring rate), cooperators are outpaced by defectors in the arms race of detaching and attaching links. Even though cooperators can swiftly break the connections with defectors during the initial few rounds, they simply run short of the opportunity necessary to cut all links to defectors in later rounds ( Fig. 4 and Supplementary Figs S7 and S8 ). Hence, some conditional cooperators give up and, as they cannot cut their ties to defectors, instead reciprocate by defecting. Thus, the overall cooperation in the group is compromised at high rewiring rates. Moreover, it is worth noting that there is a type of permanent or parasitic defector who intends to take advantage of cooperators from the very beginning. These defectors, who appear to be unaffected by losing ties (see Supplementary Fig. S9 ), have an adverse role in reducing cooperation at very high rewiring rates. In our experiments, a certain number of subjects stick with defection no matter how their neighbours respond. When cooperators run short of the opportunities to detach, defection starts spreading from these subjects having this parasitic strategy to those individuals who are conditional cooperators. In light of this, we might have observed different results if subjects had the means (for example, information) to discriminate reciprocal defection from an immutable, permanent sort of defection. This tug-of-war is a result of the fact that, in our experiment, we permit unilateral link formation; if bilateral link formation were used (and both parties had to agree to make, or break, a tie), our results would likely be different. Indeed, our results may be contrasted with a prior experiment that found a linear relationship between rewiring rates and cooperation but that also involved bilateral tie formation [18] . There are two main reasons for using the unilateral link formation in our work: theory verification and experimental practicality. First, our experiments were designed to verify predictions made by theoretical studies, which most often assume unilateral partner choice. Second, using bilateral link formation makes it difficult to keep participants in a game; such experiments often suffer from time-out issues because participants need to make each decision for every attempted partnership, in particular when the rewiring rate is high [18] . However, by using unilateral choice, participants can make decisions easily and quickly and, in contrast to experiments requiring bilateral decision making, participants rarely drop out in the middle of a session (see Supplementary Fig. S10 ). Since, in most real circumstances, people form new partnerships via mutual consent, partner-searching strategies are another area that needs to be further investigated. Nevertheless, to circumvent these difficulties, in our experimental setup, potential new ties were formed via random matching. Cooperators, if they are asked to determine whether to form a new link, could still condition their choice on the past behaviour of potential partners, and defectors had opportunities to chase after cooperators. From this point of view, our work examines how cooperation can be sustained through a tug-of-war of attachment and detachment. This tug-of-war-like process also has a substantial impact on the topological features of the emergent partner networks. We find that higher rewiring rates result in higher ultimate degree, and that cooperators have more central network positions than defectors in all experimental regimes (see Supplementary Fig. S6 ). Our experimental setup differs from this prior experiment [18] in other ways that may have affected the results, beyond the necessity of bilateral tie formation. For example, in that experiment, the 108 experimental subjects were allowed to participate in multiple sessions; thus, a learning effect across trials could be a confounder of the results; in our experiments, we restrict subjects to only one session, thus minimizing or eliminating any such learning effect. Cutting ties to defectors in dynamic networks can be seen as a form of social punishment. This is a different approach than conventional costly punishment (in which the punisher pays a cost to punish the target) that is often explored in such studies, as it does not involve explicit costs. Still, similar to tit-for-tat in repeated prisoner’s dilemma games, this sort of social punishment based on dynamic linking may have an impact by inducing people who have their ties cut to cooperate in later rounds ( Fig. 5c ). Allowing individuals to punish defectors (even when it is costly to the punisher) can promote cooperation [31] , [32] , [33] , [34] , [35] , [36] , but it reduces the payoffs of both parties and can be used against cooperators as well as defectors [37] , [38] , [39] , [40] , [41] , [42] , [43] . Cutting ties, on the other hand, is not costly when used against defectors and it is not typically used against cooperators, which makes it an attractive alternative means of maintaining cooperation. These types of experiments, on this scale, would be very hard to conduct offline [19] , [44] , [45] , and thus our work also illustrates a broader movement to develop methods to conduct experiments online [11] , [21] , [22] , [23] . Moreover, the deployment of standardized software tools affords the advantages of allowing rapid replication of results such as ours, and furthermore affords the opportunity to explore how changes in the experimental setup or the relevant parameters might affect the outcome in ways that are practically or theoretically informative. Finally, our dynamic network experiments are also related to experiments with ostracism [45] , [46] , [47] , which allow groups to use various voting systems to punish individuals by ejecting them from the group. However, in our experiments, breaking links represents a form of decentralized ostracism, where participants make their own decisions about whom to exclude from the benefits of individual cooperation. Our experiments suggest that ostracism need not be coordinated to be effective, but there may be constraints in social systems that are required to make it work. In particular, it may be important to constrain the rate at which people choose whether or not to maintain relationships to maximize the likelihood that cooperation can endure. Our findings have implications for how one might approach the formation or management of online or offline groups. Permitting or fostering intermediate rates of partner choice may be key to sustaining cooperation (or other properties, such as engagement) in groups or may be related to the ability of groups to evince other desirable traits, such as smoking cessation in online quit networks [48] or cooperation or innovation in networks of employees in workplaces [49] . Network rewiring may even be crucial to the continued existence of groups [50] . In sum, allowing individuals to dynamically update their social network connections can stabilize cooperation in large groups where cooperation is difficult to maintain solely through traditional reciprocation via changes in cooperative behaviour— but only up to a point. Social institutions that create inertia in social ties may, in fact, act to support cooperation by reducing the extent to which rewiring is possible in circumstances in which social interactions are overly fluid. Recruitment procedure A total of 1,529 subjects participated in our incentivized economic game experiments. Subjects were recruited using Amazon Mechanical Turk (MTurk) [21] , [24] , [25] , [26] , [27] , [28] . MTurk is an online labour market in which employers contract with workers to complete short tasks for relatively small amounts of money. Workers often receive a baseline payment, plus an additional bonus depending on their performance. Thus, incentivized experiments are easy to conduct using MTurk: the baseline payment corresponds to the traditional ‘show-up fee’ and the bonus payment is determined by the number of points earned during the experimental session. A number of recent studies have demonstrated the validity of behavioural experiment data gathered using MTurk. Most pertinent to our study are two direct replications using economic games. The first shows quantitative agreement in contribution behaviour in a repeated public goods game between experiments conducted in the physical lab and those conducted using MTurk with approximately tenfold lower stakes [27] . The second replication again found quantitative agreement between the lab and MTurk, with respect to cooperation in a one-shot Prisoner’s Dilemma [21] . It has also been shown that MTurk subjects are as attentive as undergraduates [26] , consistent in their answers to a range of survey questions [24] , [25] , [27] , and significantly more nationally representative [24] , and that a range of classic psychological manipulations and biases are apparent among MTurk subjects [21] , [24] . Experimental setup Our participants interacted anonymously over the internet using customized software playable in a browser window [20] . Subjects were not allowed to participate in more than one session of the experiment. In all, 90 sessions were conducted from January to April 2012. To clearly observe the effects of different rewiring rates while keeping other initial conditions the same, we completed ten sessions for each rewiring rate according to the following thresholds: network size is >10, retention rate is >75% and initial cooperative subject percentage was between 40% and 85%. As a result, 90 sessions were completed, with an average of 17.0 participants at the start of each session. Each session lasted ~1.5 h on average. The game lasted 15 rounds, but subjects were not told this, and the game ending was sudden. In each session, the subjects were paid a $3 show-up fee; each subject’s final score summed over all rounds was converted into dollars at an exchange rate of $1=1,000 points. This research was approved by the Harvard University Committee on the Use of Human Subjects. The initial environment consisted of a countdown timer of 20 min. When this time had elapsed, a ‘Go’ button became visible and the participants were required to click it to participate. Upon clicking, subjects were taken to a website external to MTurk, designed for the experiments. For each experiment, each subject was asked to take a tutorial after which the actual game would begin. If a subject did not click ‘Go’ and enter our customized website within 40 s, they were dropped from the game. If they did not complete the tutorial within 420 s, they were dropped. After 420 s of the tutorial beginning, all participants who completed the tutorial began the game. At any point during the game, if a subject was inactive for 20 s they were warned about being dropped. If they still remained inactive after 40 s, they were dropped. Only 152 out of 1,529 total subjects were dropped at some point after beginning their games and the dropout rate did not vary significantly across different rewiring rates except for 0%, which had a lower dropout rate ( Supplementary Fig. S10 ). Statistical model of cooperation and density change Analysing the data from our experiment (for example, Supplementary Fig. S3 ) requires more than an analysis of mere average values. For instance, the average values by round do not represent directly the slopes of the change through a session. Moreover, ratio data represented as the cooperation rate, which is limited to be between 0 and 1, does not come from a population that is normally distributed. In addition, multiple observations from the same subject and observations from multiple subjects within the same session are not independent. Thus, we need to deal with the nested structure of errors in our statistical analysis. Hence, we used a statistical analysis based on a GLMM involving logistic regression with nested random effects [30] . GLMM estimates coefficients in the linear predictor and random effects, which comes from individual differences, at the same time, using the maximum-likelihood methods. To be concrete, here is how the model was implemented to get the statistical results on strategy selection in Fig. 2 : let p i,w denote the probability of player i selecting cooperation in the session with rewiring rate w ; let x be the round number of the session; and let γ 0,i , γ 1,i denote the random effects nested within the experimental session player i belongs to. Then, we have In the terminology of GLMM, equation (1) is called the ‘link function’ and equation (2) is termed the ‘linear predictor.’ Here, we used a logistic function as the link function because the response variable p is assumed to obey the binominal distribution. The random effects γ can be approximated by the normal distribution with mean value zero. Using maximum-likelihood methods to minimize the random error e , we then estimated the β coefficients that represent the fixed effect of the rewiring rate w. In this way, the model allows us to estimate the β coefficients in the linear predictor while taking into account random effects due to individual variation. All analysis was performed using R version 2.14.1. We calculated the probability of subjects selecting cooperation by round using the foregoing model. The estimated values are shown in Supplementary Table S1 . Figure 2 showed the coefficients β 1 in Supplementary Table S1 as a level of cooperation change. From the statistical model, we see that the dependence of cooperation on the rewiring rate is not monotonic but shows a peak around a 70% rewiring rate. It is not appropriate to estimate the levels of density change across all rounds, because the changing rate is not time dependent ( Supplementary Fig. S4 ). For instance, at high rewiring rates the density dramatically increases in the initial rounds and then stays roughly constant. We call the former the ‘pre-stable state’ and the later the ‘stable state’. We determined the number of rounds needed to transition from the pre-stable and the stable state for each rewiring rate. The method is to apply GLMM with logistic regression by group of three or four consecutive rounds. The results are shown in Supplementary Table S2 . When the estimated slope is not significantly different compared with the first set, we concluded that the network had reached the stable state. The critical number of rounds for different rewiring rates is shown in Supplementary Fig. S5 . We see that the density reaches the stable state faster with increasing rewiring rate. Statistical model of reciprocity Each subject has to make a choice between cooperation and defection every round. Subjects are informed of previous strategies of their neighbours at this time. Figure 5a shows that the previous strategies of neighbours affect the future choice of the focal player. The lines in Fig. 5a are probability functions P ( μ ) estimated by GLMM incorporating random effects for sessions and individuals. P ( μ ) is a logistic function where μ is the ratio of cooperative players among neighbours (the terms of the random effects are omitted in the equation (3) for clarity). The estimated fixed effects coefficients for changing from cooperation to defection are β 1 =2.06 and β 2 =−4.94, and those for changing from defection to cooperation are β 1 =−2.15 and β 2 =2.50. Using the estimated coefficients, we can calculate the threshold level of cooperation among neighbours such that average subjects switch strategy with 50% chance by From equation (4), subjects change from cooperation to defection with 50% chance when μ is 41.7% and from defection to cooperation when μ is 86.0%. Cooperators are less likely to remain cooperative with increasing numbers of neighbours who defected. On the other hand, defectors are more likely to change their strategy with an increasing cooperation level among their neighbours. These phenomena are called ‘strategy reciprocity’, and they contribute to a cascade of cooperation or defection in the static network. A subject’s decision can influence the whole network by affecting the cooperation probability of his neighbours. Notably, the probability of cooperators changing into defectors is, on average, higher and more sensitive to the cooperativity of neighbours than that of defectors changing to cooperators. This means defection is favoured over cooperation (if subjects do not also have opportunities to change their neighbours). How to cite this article: Shirado, H. et al. Quality versus quantity of social ties in experimental cooperative networks. Nat. Commun. 4:2814 doi: 10.1038/ncomms3814 (2013).